Variant Plateau’s law in atomically thin transition metal dichalcogenide dome networks 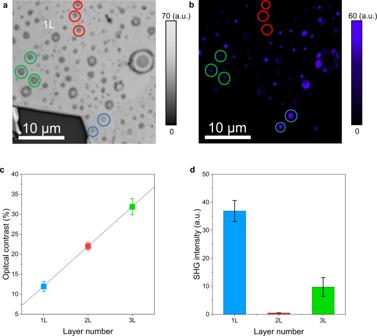Fig. 1: Optical characterisation of mono- and few-layer pressurised nano-domes in TMDs. a, Optical microscope image of pressurised domes generated on a WS2flake, whereby mono- (1 L), bi- (2 L) and tri-layer (3 L) domes have been highlighted by blue, red and green circles, respectively. The layer number of the dome is initially identified from the optical contrast.bSecond harmonic generation (SHG) mapping of the same flake shown ina. 1 L domes show the strongest SHG signal, whilst 2 L domes are almost invisible under the same excitation and collection conditions.cMeasured optical contrast as a function of dome layer number. The measured optical contrast for 1–3 L domes with similar sizes are 11.9% ± 1.3% (blue), 22.0% ± 0.9% (red) and 31.9% ± 2.0% (green), respectively. The error bars represent statistical variation from at least 4 domes for each group with different layer number.dMeasured SHG intensity as a function of layer number of the domes. The measured SHG intensities for 1–3 L domes with similar sizes are 36.93 ± 3.74, 0.54 ± 0.01 and 9.79 ± 3.36 arbitrary unit (a.u.), represented by blue, red and green bars, respectively. The error bars represent statistical variation from at least 5 domes from each group with different layer number. Since its fundamental inception from soap bubbles, Plateau’s law has sparked extensive research in equilibrated states. However, most studies primarily relied on liquids, foams or cellular structures, whereas its applicability has yet to be explored in nano-scale solid films. Here, we observed a variant Plateau’s law in networks of atomically thin domes made of solid two-dimensional (2D) transition metal dichalcogenides (TMDs). Discrete layer-dependent van der Waals (vdWs) interaction energies were experimentally and theoretically obtained for domes protruding in different TMD layers. Significant surface tension differences from layer-dependent vdWs interaction energies manifest in a variant of this fundamental law. The equivalent surface tension ranges from 2.4 to 3.6 N/m, around two orders of magnitude greater than conventional liquid films, enabling domes to sustain high gas pressure and exist in a fundamentally variant nature for several years. Our findings pave the way towards exploring variant discretised states with applications in opto-electro-mechanical devices. Since Joseph Plateau’s fundamental observations [1] of soap bubbles in the 19th century revealed their borders meet at equal joint angles of 120°, this law has been a prominent physical law in natural science. Apart from soap bubbles [1] , [2] , [3] , [4] , [5] , [6] , Plateau’s law naturally occurs in liquid foams such as beer froth, and in solid foams such as cells, honeycombs and metallic foams [7] , [8] , [9] , [10] . Even in emerging two-dimensional (2D) materials such as graphene [11] , the atomic arrangement of carbon atoms form a hexagonal structure at 120° to assume an equilibrated state [12] . Whilst some studies have shown that the joint angles in bubbles and foams are not always 120°, the angle deviation is quite small of only a few degrees [13] , [14] , [15] , [16] . Due to the low surface tension ( σ ) of liquids, such as 0.07–0.09 N/m for water [17] and 0.025 N/m for soap bubbles [18] , the capped pressure in liquid bubbles is low and they only exist for short periods of time before bursting. On the other hand, atomically thin layered materials such as graphene [11] and transitional metal dichalcogenides (TMDs) [19] , [20] are becoming promising candidate materials for the creation of nano-bubbles [21] , [22] , [23] , [24] , [25] , [26] . These 2D mono- and few-layer [27] , [28] materials are at least two orders of magnitude thinner than soap bubble films [29] , but have shown strong mechanical strength [30] , [31] , high resistance to common alkaline and acids [32] , [33] , as well as fabulous chemical and thermal stability [34] . All previously demonstrated nano-bubbles in 2D materials were isolated singular ones without networking topologies [21] , [22] , [23] , [24] , [25] . Herein, we successfully created atomically thin TMD dome networks and observed variant Plateau’s law in nano-scale solid systems. Variant Plateau’s law is due to thickness dependent interlayer adhesion energy between the first few interacting TMD layers and the basal plane, causing thickness dependent stiffness values depending on dome layer number, resulting in large effective surface tension differences, which leads to the formation of large joint angle differences of approximately 77° between the largest and smallest angles. Results contrast with the commonly observed equal joint angles and 0° angle difference commonly associated with Plateau’s law, demonstrating that this variant is observed due to our 2D TMD dome networks. Generation and characterisations of TMD pressurised domes Recently, we successfully used a low-energy (<15 eV) proton irradiation technique to produce pressurised and spherical monolayer hydrogen domes on the surface of bulk TMDs [25] . Here, we increased the proton beam energy to ~25 eV, which allowed protons to deliberately penetrate deeper basal planes of the TMD, leading to the creation of mono-(1 L), bi-(2 L), and tri-layer (3 L) pressurised hydrogen nano-domes (Fig. 1 ). Dome layer number was initially identified from optical contrast (Fig. 1a ) and further confirmed by second harmonic generation (SHG) imaging performed on the same flake (Fig. 1b ). The optical contrast showed a linear relationship with layer number (Fig. 1c ), consistent with a previous report [35] . 1 L and 3 L domes exhibit intense and less intense SHG signals, respectively, and 2 L domes show no SHG (Fig. 1d ), which is attributed to the fact that for 2H phase TMDs, broken inversion symmetry only exits in samples with odd layer number [36] , [37] . The percentage yield of 2 L and 3 L domes was enhanced under higher proton dosage, obtained via statistical analysis (Supplementary Fig. 1 ). Fig. 1: Optical characterisation of mono- and few-layer pressurised nano-domes in TMDs. a , Optical microscope image of pressurised domes generated on a WS 2 flake, whereby mono- (1 L), bi- (2 L) and tri-layer (3 L) domes have been highlighted by blue, red and green circles, respectively. The layer number of the dome is initially identified from the optical contrast. b Second harmonic generation (SHG) mapping of the same flake shown in a . 1 L domes show the strongest SHG signal, whilst 2 L domes are almost invisible under the same excitation and collection conditions. c Measured optical contrast as a function of dome layer number. The measured optical contrast for 1–3 L domes with similar sizes are 11.9% ± 1.3% (blue), 22.0% ± 0.9% (red) and 31.9% ± 2.0% (green), respectively. The error bars represent statistical variation from at least 4 domes for each group with different layer number. d Measured SHG intensity as a function of layer number of the domes. The measured SHG intensities for 1–3 L domes with similar sizes are 36.93 ± 3.74, 0.54 ± 0.01 and 9.79 ± 3.36 arbitrary unit (a.u. ), represented by blue, red and green bars, respectively. The error bars represent statistical variation from at least 5 domes from each group with different layer number. Full size image Due to the resolution limit of conventional optical microscopes, distinguishing the layer number of small-sized domes is challenging. Therefore, AFM height imaging (Fig. 2a–c ) and stiffness mapping images of the domes were obtained and used to depict the layer dependent mechanical properties (Fig. 2d–f ). Given the sample domes’ similar radii (500–630 nm), the obtained stiffness images reveal a substantial relationship between layer number and mechanical properties. An inferred method based on a strong boundary condition (detailed in Supplementary Note 1 ) [38] , [39] was used to calculate the 2D modulus ( E 2D ) of the domes formed in different layers. Finite element analysis (FEA) (Supplementary Note 2 ) was compared against the experimental data for the nano-indentation process using the derived E 2D , illustrating good agreement (Fig. 2g ). The measured stiffness showed a maximum value at the dome centre and decreased gradually by 20–30% as the AFM tip moved away from centre to the edge, which also matched with simulation results from FEA and analytically (Supplementary Fig. 2 ). During indentation, there should be a resultant backward pressure applied due to the internal pressure encapsulated by a dome, and this may explain slight discrepancies [38] , [39] ; however, overall, this does not appear to be a major influence as the FEA accounts for both pressures and a good agreement is found at the centre of domes. Slight discrepancies arise when moving away from the dome centre, which may be due to the non-uniform pressure distribution acting on the nano-indenter due to dome curvature. Moreover, the measured stiffness (at the dome centre) of different 1 L, 2 L and 3 L domes exhibit an exponentially decaying trend with increasing dome radius for a constant E 2D , which agrees well with the FEA simulation as shown in Fig. 2h . FEA was also conducted for slightly modified dome footprint shapes which showed comparable stiffness values with a perfect circular dome footprint (Supplementary Fig. 3 and Supplementary Note 3 ). The gas pressure of domes also possess an exponential trend, leading to higher pressure up to tens of MPa capped in smaller and stiffer domes (see Supplementary Fig. 4 ). Moreover, we could estimate the pressure of domes at low T to verify the inferred method against the phase transition of H 2 molecules, showing good agreement as in Supplementary Fig. 5 and Supplementary Note 4 . Fig. 2: Mechanical characterisations of mono- and few-layer pressurised TMD nano-domes. a – c Atomic force microscope (AFM) images of a 1 L ( a ), 2 L ( b ) and 3 L dome ( c ). The measured centre dome height ( h m ) to radius ( R ) ratio ( h m /R ) for 1–3 L domes are 0.18, 0.17, and 0.16, respectively. d – f Stiffness mapping images measured for the 1–3 L domes shown in a – c . g Force-indentation curves (dots) measured at the centre of domes with different layer numbers (1–3 L). The simulated force-indentation curves (solid lines) from finite element analysis (FEA) match very well with the measured ones. The inset shows the experimental set up for data acquisition: an AFM tip was used for the mechanical nano-indentation of domes. h Measured stiffness as a function of dome radius (solid dots), for 1–3 L domes. Simulated results (lines) by FEA match well with experimental observations. i Extracted two-dimensional modulus ( E 2D ) of WS 2 as a function of layer number. The extracted E 2D values are 244.0 ± 35.7, 429.5 ± 37.7 and 520.4 ± 49.2 N/m for 1–3 L WS 2 domes, respectively. The error bars represent statistical variation from 20 domes for each group with different layer number. Full size image Thus, using layer-dependent stiffness curves and dome radius, we can quickly identify thickness and mechanical properties of domes that match well with FEA (Fig. 2g, h ). 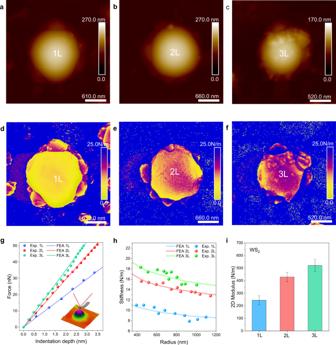Fig. 2: Mechanical characterisations of mono- and few-layer pressurised TMD nano-domes. a–cAtomic force microscope (AFM) images of a 1 L (a), 2 L (b) and 3 L dome (c). The measured centre dome height (hm) to radius (R) ratio (hm/R) for 1–3 L domes are 0.18, 0.17, and 0.16, respectively.d–fStiffness mapping images measured for the 1–3 L domes shown ina–c.gForce-indentation curves (dots) measured at the centre of domes with different layer numbers (1–3 L). The simulated force-indentation curves (solid lines) from finite element analysis (FEA) match very well with the measured ones. The inset shows the experimental set up for data acquisition: an AFM tip was used for the mechanical nano-indentation of domes.hMeasured stiffness as a function of dome radius (solid dots), for 1–3 L domes. Simulated results (lines) by FEA match well with experimental observations.iExtracted two-dimensional modulus (E2D) of WS2as a function of layer number. The extractedE2Dvalues are 244.0 ± 35.7, 429.5 ± 37.7 and 520.4 ± 49.2 N/m for 1–3 L WS2domes, respectively. The error bars represent statistical variation from 20 domes for each group with different layer number. Figure 2i reveals that the 2D modulus monolithically increases with layer number for 1–3 L WS 2 domes, consistent with the trend reported for suspended membranes [30] . Similarly, we also used the inferred indentation method to experimentally obtain the 2D modulus of MoS 2 domes shown in Supplementary Fig. 6a . Resolving layer-dependent adhesion energies in TMDs by domes The vdW adhesion energy ( γ ) plays an important role in layered materials and their physical properties, and several techniques have been reported to measure the adhesion energy between monolayer materials and the substrate [40] , [41] , [42] , [43] , [44] , γ in this work refers to the interlayer adhesion between TMD basal planes from the remaining bulk flake and not the base substrate. The adhesion energies in layered materials should be layer dependent, particularly for mono- and few-layer domain structures, but this layer-dependence was not previously explored. Here, our 1 L, 2 L, and 3 L domes provide a fascinating platform to probe the intrinsic and discrete layer-dependent adhesion energies in TMDs. We firstly used density functional theory (DFT) (Supplementary Note 5 ) to calculate the γ values for 1 L WS 2 at 0 and 300 K (Fig. 3a ). The calculated γ value at 0 K is consistent with previously reported values [45] ; the calculated γ value at 300 K is ~50% higher than that at 0 K, consistent with recent results from experiments that γ is enhanced at higher temperature [40] . The γ values for 1 L, 2 L and 3 L WS 2 were experimentally determined based on the material properties of the nano-domes (Supplementary Note 1 ), which showed a clear layer-dependence, matching well with our DFT calculated values at 300 K, including the presence of trapped hydrogen molecules (Fig. 3b ). Minor differences may be attributed to two reasons; the first being the variation in the bond length of the topmost layers and inter-layer spacing induced by the external pressure, and thermal effects in ambient conditions [46] . Another reason may be modulated mechanical properties caused by trapped hydrogen molecules [47] . DFT results revealed that adsorbed hydrogen molecules affect the 2D modulus of monolayer TMDs, but have a small effect in few layer TMDs (Supplementary Fig. 7 ). This explains the larger discrepancy between experimental values of adhesion energy and DFT calculated values in monolayer domes, whereas few layer domes have negligible difference. Similarly, the experimental γ values for 1 L, 2 L and 3 L MoS 2 are discrete and layer-dependent (Supplementary Fig. 6b ). Our γ values for TMD monolayers (Fig. 3b and Supplementary Fig. 6b ) are consistent with previously reported experimental results [40] . Fig. 3: Resolving layer-dependent adhesion energies in TMDs by nano-domes. a Calculated energy required to separate a WS 2 monolayer from the bulk as a function of separation distance ( d ), by DFT (dots) and analytical solution (line), at 0 (blue) and 300 K (red). d 0 is the initial separation distance. The adhesion energy is defined to be the energy per area required to separate the layer from the bulk. The adhesion energies of a WS 2 monolayer at 0 and 300 K are calculated to be 21.5 and 29.7 meV/Å 2 , respectively. The analytical solution has the form \({{{{{{\rm{\gamma }}}}}}}_{{dist}}=\,{{{{{\rm{\gamma }}}}}}\left[\frac{3}{2}{(\frac{{d}_{0}}{d})}^{3}-\frac{1}{2}{(\frac{{d}_{0}}{d})}^{9}\right]\) , where γ dist is the monolayer-surface interaction energy per unit area at a corresponding separation distance and γ is the interfacial adhesion energy per unit area [45] ; The inset provides the schematic illustration of the initial interlayer distance ( d 0 ) and modified separation distance ( d ) in WS 2 . b Measured layer-dependent adhesion energies of WS 2 , which are the energies required to exfoliate top layers (1–3 L) from a WS 2 bulk flake, using nano-domes. The adhesion energy values obtained from 1–3 L WS 2 are 33.8 ± 3.0, 42.6 ± 2.5 and 45.0 ± 4.2 meV/Å 2 , all of which are in good agreement with the DFT results of 31.5, 40.3 and 43.5 meV/Å 2 , respectively. The error bars represent statistical variation from 20 domes for each group with different layer number. Full size image Identification of joint bi-dome structure and configurations When the exfoliated TMD thick flake is exposed to ~25 eV proton irradiation, hydrogen protons penetrate the top few basal planes of the bulk TMD flake, and then reduce to form hydrogen molecules accumulated in the top few TMD layers, forming mono- and few-layer domes (Fig. 4 a Stage I-II). With longer proton exposure time, the domes grow and interface with each other, and the inner pressure from the 1 L dome (on the right) overcomes the vdWs adhesion force and lifts off the top-most layer partially covering the adjacent 2 L dome (on the left), eventually forming a joint double dome (bi-dome) system (Fig. 4 a Stage III-V). Therefore, the hydrogen molecules in our 1 L, 2 L and 3 L domes exist in different basal planes of the TMD, leading to intriguing different joint dome configurations and interaction dynamics among domes. It is important to note here that the substrate is the TMD flake beneath the resulting domes and not the base SiO 2 /Si substrate, as growing domes on different base substrates still results in a universal height to radius ratio [25] . Experimentally, many different coalescing dome formations were observed, and the most common case was the bi-dome presented in the AFM image as shown in Fig. 4b . This case is the existence of a bi-dome composed of a large 1 L dome coinciding with a smaller 2 L dome, demonstrating complex interaction between hydrogen accumulation underneath different basal planes of the TMD. To maintain stability, domes sharing common vertices must be in different layers of the TMD; otherwise, domes will merge resulting in larger domes in the same basal plane to minimise their surface energy, analogous to liquid bubbles. The structure and configuration of a joint bi-dome was directly confirmed by a bursting experiment test (Supplementary Fig. 8 and Supplementary Note 6 ). To further characterise the structure and confirm the configuration, stiffness mapping was conducted among the joint domes and a clear dependency between the stiffness of interacting domes was observed (Fig. 4c ). This reaffirms domes are in different layers as illustrated by the inset in Fig. 4c , where the smaller 2 L dome exhibits much higher stiffness than the larger 1 L dome. FEA simulations of the generated height profile and stiffness of the two merging domes (with configuration depicted by the inset in Fig. 4c ) is given in Fig. 4d, e , respectively, illustrating good agreement between the simulation and experimental results. Some discrepancies near the transition region are visible, which is attributable to the AFM resolution or a mismatch in modelling the geometry and boundary conditions. This demonstrates that domes function as highly pressurised membranes with high tension across the dome interface between internal and external pressures (Supplementary Note 7 ). Moreover, a very sharp stiffness transition edge between dome layers is visible (Fig. 4e ), further confirming the two domes are sitting in different basal planes. The same method was applied to a different joint configuration with a larger 2 L region and smaller 1 L region, also showing good agreement between simulation and experiment (Supplementary Fig. 9 ). Fig. 4: Identification of structure configuration of a joint bi-dome via nano-indention. a Schematic illustration of a joint bi-dome formation process. b AFM image of a WS 2 joint bi-dome made of a large 1 L dome and small 2 L dome. c Stiffness mapping of the joint bi-dome shown in a . The inset indicates the structure of the domes along the white dashed line in b . d Measured height profile (grey) of the joint bi-dome along the white dashed line shown in b . The simulated profile (red) generated by FEA reasonably matches with the measured one. e Measured stiffness (solid blue dots) as a function of scan distance along the white dashed line shown in b . Simulated stiffness values by FEA calculation (red diamond) match well with experimental values. The sharp drop of stiffness value at 300 nm corresponds to the joint boundary between 2 L and 1 L domes. Full size image Observation of variant Plateau’s law in joint dome systems In a bi-dome system, three joint angles between adjoining edges were formed, termed as α 1 , α 2 and α 3 (inset in Fig. 5a ). The values of α 1 , α 2 and α 3 for WS 2 bi-domes were measured to be 153.1° ± 8.8°, 75.6° ± 9.8° and 131.2° ± 6.1°, respectively (Fig. 5a ), differing with each other, which is in great contrast to Plateau’s law of equal joint angles of 120° as observed in soap bubbles [1] . The values of α 1 , α 2 and α 3 for WS 2 bi-domes were calculated (Supplementary Note 8 and Supplementary Fig. 10 ) to be 152.6°, 72.3° and 135.1°, respectively, agreeing well with the experimental values (Fig. 5a ). A large difference of ~77.5° between α 1 and α 2 was observed in WS 2 bi-dome systems, such large deviation has not been previously reported, demonstrating a variant Plateau’s law. The governing reason for this behaviour is due to the large unequal effective surface tension ( σ ) differences in the different dome layers, where 1 L, 2 L and 3 L domes have experimental σ values of 2.4 ± 0.3, 3.5 ± 0.3, 3.6 ± 0.3 N/m, respectively, which is significantly higher than other systems (Supplementary Note 8 ). The large difference among the σ values of 1 L, 2 L and 3 L domes is a direct result of the discrete nature of γ in 1–3 L TMDs as shown in Fig. 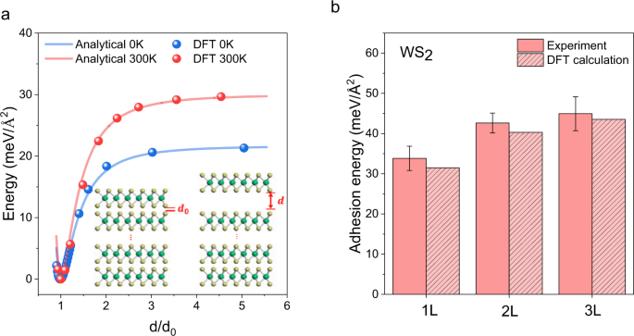Fig. 3: Resolving layer-dependent adhesion energies in TMDs by nano-domes. aCalculated energy required to separate a WS2monolayer from the bulk as a function of separation distance (d), by DFT (dots) and analytical solution (line), at 0 (blue) and 300 K (red).d0is the initial separation distance. The adhesion energy is defined to be the energy per area required to separate the layer from the bulk. The adhesion energies of a WS2monolayer at 0 and 300 K are calculated to be 21.5 and 29.7 meV/Å2, respectively. The analytical solution has the form\({{{{{{\rm{\gamma }}}}}}}_{{dist}}=\,{{{{{\rm{\gamma }}}}}}\left[\frac{3}{2}{(\frac{{d}_{0}}{d})}^{3}-\frac{1}{2}{(\frac{{d}_{0}}{d})}^{9}\right]\), whereγdistis the monolayer-surface interaction energy per unit area at a corresponding separation distance andγis the interfacial adhesion energy per unit area45; The inset provides the schematic illustration of the initial interlayer distance (d0) and modified separation distance (d) in WS2.bMeasured layer-dependent adhesion energies of WS2, which are the energies required to exfoliate top layers (1–3 L) from a WS2bulk flake, using nano-domes. The adhesion energy values obtained from 1–3 L WS2are 33.8 ± 3.0, 42.6 ± 2.5 and 45.0 ± 4.2 meV/Å2, all of which are in good agreement with the DFT results of 31.5, 40.3 and 43.5 meV/Å2, respectively. The error bars represent statistical variation from 20 domes for each group with different layer number. 3b . Additionally, some domes in this work are partially sitting on top of others; the dome part sitting on top of another dome has different γ compared to the part being exfoliated from the bulk flake. For example, it requires less energy to detach a 1 L sheet from a 2 L sheet, rather than from the bulk (Supplementary Fig. 10b ). Domes merging in this manner demonstrate the discrete nature of γ , leading to significant variations in the effective σ of each dome. Similarly, large variations of the joint angles were also observed and analytically calculated for MoS 2 , demonstrating excellent agreement (Supplementary Fig. 11a ). Fig. 5: Observation of variant Plateau’s law in bi- and tri-dome systems. a Histogram of the joint angles ( α i , i = 1, 2, 3) in WS 2 bi-dome systems, extracted experimentally (solid bars) and analytically (patterned bars). The inset shows the angle notations in a standard bi-dome configuration. The experimental values for joint angle are 153.1° ± 8.8°, 75.6° ± 9.8° and 131.2° ± 6.1° for α 1 , α 2 and α 3, respectively. Statistical data was collected from 20 joint bi-domes. The calculated values for α 1 , α 2 and α 3, are 152.6°, 72.3° and 135.1°, respectively, all of which are in good agreement with experimental values. b Histogram of the joint angles ( β i , i = 1, 2, 3) in WS 2 tri-dome systems, extracted experimentally. The inset shows the angle notations in a standard tri-dome configuration. The experimental values for joint angle are 135.5° ± 6.4°, 104.6° ± 7.1° and 119.9° ± 3.7° for β 1 , β 2 and β 3 , respectively. Statistical data was collected from 15 joint tri-domes. c AFM image of a WS 2 tri-dome system, consisting of 1 L, 2 L and 3 L domes joint together. d Stiffness mapping image of tri-dome shown in c . The layer-dependent stiffness can be clearly distinguished. Full size image To exacerbate the large deviations from Plateau’s law in TMD domes, the joint angles β 1, β 2 and β 3 of WS 2 tri-dome systems were also experimentally determined as shown in Fig. 5b–d . The values of β 1, β 2 and β 3 for WS 2 tri-domes were measured to be 135.5° ± 6.4°, 104.6° ± 7.1° and 119.9° ± 3.7°, respectively, also clearly demonstrating variant Plateau’s law, whereby joint angles no longer merge at 120°. Similar large angle deviations were also observed in MoS 2 tri-domes (Supplementary Fig. 11b ). The largest angle was found in the 1 L region in a tri-dome system, similar to that observed in a bi-dome system; the angle difference ( β 1 - β 2 ) in a tri-dome system is smaller than that in a bi-dome system ( α 1 - α 2 ). A statistical analysis of angle variation in WS 2 and MoS 2 bi-dome and tri-dome networks (Fig. 5a, b , and Supplementary Fig. 11 ) concluded that α 1 and β 1 for both material systems (WS 2 and MoS 2 ) are the largest among all three angles. Moreover, bi-dome systems have larger angle deviation compared to tri-dome systems. The α 1 , α 2 and α 3 of a WS 2 bi-dome system deviate by 8.8°, 9.8° and 6.1°, respectively, whilst β 1 , β 2 and β 3 exhibit lower deviations of 6.4°, 7.1° and 3.7°, respectively. This could be attributed to the fact that bi-domes are more likely to be influenced by the surrounding conditions on the bulk flake, including side domes, surface contaminants and surface topology, leading to larger deviation in joint angles α . Owing to a trigonal structure in tri-dome systems, a better structural stability generates smaller deviation in joint angles compared to bi-domes, and WS 2 and MoS 2 tri-dome systems have comparable angle values for β 1 , β 2 and β 3 . In addition, it is worth to note that the validity of the variant of Plateau’s law in complex dome network systems. To prove this, we characterised a one-dimensional (1D) dome chain and 2D superlattice structure with bi-dome and tri-domes as the repeating unit (Supplementary Fig. 12 ). In the 1D dome chain, it also proves that the largest and smallest angles are α 1 in 1 L regions and α 2 in 2 L regions, respectively, which is confirmed by stiffness mapping (Supplementary Fig. 12b ). This reaffirms that the variations in joint angles, regardless of the complexity of the network structure, are induced by layer-dependent mechanical properties including E 2D , γ and σ . Furthermore, due to the robustness of TMDs, E 2D and γ remain constant over time, allowing the morphological structure and joint angles to endure for a long period without variations (Supplementary Fig. 13 ), even in the presence of external stimuli (nano-indentation and optical tests). This means determination of joint angles of the network is a reliable tool to quickly identify layer number of domes in a network, exemplified by the 2D dome network shown in Supplementary Fig. 12c . We successfully fabricated 1 L, 2 L and 3 L pressurised hydrogen nano-domes, and their networks, using low-energy proton irradiation on TMD flakes. Dome layer number was identified and confirmed by optical contrast, SHG imaging and high-resolution stiffness mapping. The layer-dependent mechanical properties of domes revealed by AFM nano-indentation match well with FEA simulations. 1–3 L domes provide a fascinating platform for resolving the discrete layer-dependent adhesion energies in TMDs, which matched with DFT calculations. Joint bi-dome and tri-dome systems were formed when the domes sitting in different basal planes grew and interacted with each other. The layer-structure and configurations of joint domes were successfully identified and confirmed by stiffness mapping, FEA calculation and bursting test. Variant Plateau’s law was observed in bi-dome and tri-dome systems, which is due to the large variations of effective surface tension in different layer number domes, arising from the discrete vdWs adhesion energy in TMDs. For example, our bi-dome system has a large joint angle difference of more than 77°, in great contrast to conventional liquid bubble systems that have equal joint angles. Our solid domes equivalent surface tension values range from 2.4 to 3.6 N/m, which is two orders of magnitude larger than their liquid or foam counterparts enabling high pressure encapsulation. The variant Plateau’s law observed in experiments agrees with our analytical calculation. Furthermore, stable and long-lasting 1D and 2D dome networks were realised in experiments with multiple domes sitting in different basal planes of the TMD. Dome networks can become a promising topic for generating 1D or 2D nanostructures with large variation in properties enabling new device applications in the fields of nano-photonics, nano-opto-mechanics and quantum science. Fabrication of the domes Thick TMD flakes are mechanically exfoliated onto various substrates including SiO 2 /Si (275 nm SiO 2 ), Au deposited and doped silicon. The samples are subsequently placed in the chamber for proton irradiation treatment in a high vacuum condition. During the treatment, the pressure inside the chamber is P = 1.4 × 10 −4 mbar, with hydrogen gas delivered at a flow rate of 30 sccm. Meanwhile, the H + protons produced in an ionisation chamber will be accelerated and guided onto the sample surface, as a form of proton beam with energy at least 25 eV. The relative larger energy enables protons to deliberately penetrate deeper basal planes of the TMD, creating different layered domes and dome networks. The entire treatment process normally takes a few hours to complete. Optical characterisation Optical microscope images were taken by a Zeiss 780 confocal microscope equipped with a 633 nm single photon laser. SHG measurement were also performed on a Zeiss 780 confocal microscope using a Ti:Sapphire laser (150 fs, 80 MHz). The sample is excited and measured under a 50× confocal objective lens (NA = 0.85), and results are collected in the reflection mode at a fundamental laser wavelength of 900 nm. All data of optical characterisation measurements were processed and analysed by image processing software, Zen 3.2 (blue edition). AFM Nano-indentation The topographic images were captured using a Bruker Dimension Icon AFM. The aspect ratio of the domes was measured in Scanasyst mode with soft cantilevers, Scanasyst-Air, whose nominal spring constant k and nominal tip radius are 0.4 N/m and 2 nm, respectively. Using soft tips to obtain the profile and topographic information is designed to minimise tip–sample interaction and avoid modifying the shape of the domes or destroy domes. Indentation experiments on TMD domes were performed in Quantum Nano Mechanical (QNM) mode. The tips used for the measurement is RTESPA-300 with k = 40 N/m and a nominal R tip = 8 nm. Before the measurement, the tips required calibration in terms of resonance frequency, deflection sensitivity, contact area, and spring constant to ensure results are repeatable. 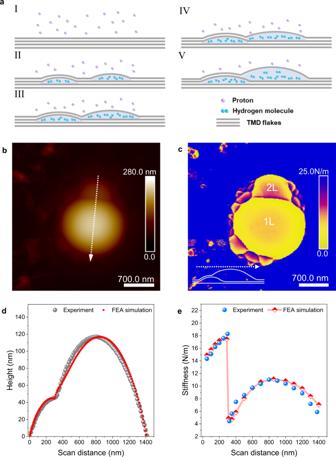Fig. 4: Identification of structure configuration of a joint bi-dome via nano-indention. aSchematic illustration of a joint bi-dome formation process.bAFM image of a WS2joint bi-dome made of a large 1 L dome and small 2 L dome.cStiffness mapping of the joint bi-dome shown ina. The inset indicates the structure of the domes along the white dashed line inb.dMeasured height profile (grey) of the joint bi-dome along the white dashed line shown inb. The simulated profile (red) generated by FEA reasonably matches with the measured one.eMeasured stiffness (solid blue dots) as a function of scan distance along the white dashed line shown inb. Simulated stiffness values by FEA calculation (red diamond) match well with experimental values. The sharp drop of stiffness value at 300 nm corresponds to the joint boundary between 2 L and 1 L domes. 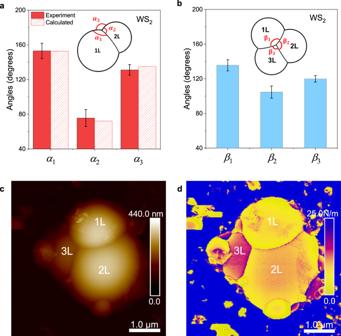Fig. 5: Observation of variant Plateau’s law in bi- and tri-dome systems. aHistogram of the joint angles (αi,i= 1, 2, 3) in WS2bi-dome systems, extracted experimentally (solid bars) and analytically (patterned bars). The inset shows the angle notations in a standard bi-dome configuration. The experimental values for joint angle are 153.1° ± 8.8°, 75.6° ± 9.8° and 131.2° ± 6.1° forα1,α2andα3,respectively. Statistical data was collected from 20 joint bi-domes. The calculated values forα1,α2andα3,are 152.6°, 72.3° and 135.1°, respectively, all of which are in good agreement with experimental values.bHistogram of the joint angles (βi, i= 1, 2, 3) in WS2tri-dome systems, extracted experimentally. The inset shows the angle notations in a standard tri-dome configuration. The experimental values for joint angle are 135.5° ± 6.4°, 104.6° ± 7.1° and 119.9° ± 3.7° forβ1,β2andβ3, respectively. Statistical data was collected from 15 joint tri-domes.cAFM image of a WS2tri-dome system, consisting of 1 L, 2 L and 3 L domes joint together.dStiffness mapping image of tri-dome shown inc. The layer-dependent stiffness can be clearly distinguished. The indentation force was adjusted and set between 50 and 100 nN to avoid the fact that large forces might destroy domes. For the force curves at different locations, they were extracted using ramp mode and this mode could record extending and extracting cycles at different locations on the dome samples. Stiffness values could be processed by calculating the slope of the loading part of extending cycles. For the adhesion energy measurement, the 2D modulus ( E 2D ) was extracted and calculated based on the force curves at the centre of the dome samples.